Rugged and breathable forms of stretchable electronics with adherent composite substrates for transcutaneous monitoring Research in stretchable electronics involves fundamental scientific topics relevant to applications with importance in human healthcare. Despite significant progress in active components, routes to mechanically robust construction are lacking. Here, we introduce materials and composite designs for thin, breathable, soft electronics that can adhere strongly to the skin, with the ability to be applied and removed hundreds of times without damaging the devices or the skin, even in regions with substantial topography and coverage of hair. The approach combines thin, ultralow modulus, cellular silicone materials with elastic, strain-limiting fabrics, to yield a compliant but rugged platform for stretchable electronics. Theoretical and experimental studies highlight the mechanics of adhesion and elastic deformation. Demonstrations include cutaneous optical, electrical and radio frequency sensors for measuring hydration state, electrophysiological activity, pulse and cerebral oximetry. Multipoint monitoring of a subject in an advanced driving simulator provides a practical example. Recent advances in stretchable electronics and sensors enable their intimate integration with the skin in ways that bypass limitations of traditional technologies [1] , [2] , [3] , [4] . These systems softly laminate onto the epidermis to yield highly functional, cutaneous interfaces that are mechanically, thermally and chemically ‘invisible’ to the user [5] , [6] with potential for use outside of hospitals and traditional laboratory settings. Opportunities in seamless, continuous assessment of health/wellness, advanced function in wound monitoring/care and human–machine control systems motivate research in this field [7] , [8] . Desirable physical attributes include a low modulus and bending stiffness with elastic mechanics for strains of tens of percent, or more, as well as a thin and lightweight layout with low thermal mass, high water and gas permeability, robust and non-invasive adhesion to the skin, even in regions with significant contours and hair, and a mechanically rugged, reusable construction. Achieving all of these features in a single system is challenging. As an example, the mechanically rugged and reusable construction tends to favour choices in materials and designs that are at odds with the other attributes. The consequences have practical importance. For instance, removing a device that is strongly bonded to the skin demands forces that can lead to large, fracture-inducing strains in thin, ultralow modulus platforms. A physically tough, high-modulus design avoids these types of failures, but does not allow soft integration with the skin. The results presented here resolve this apparently conflicting set of requirements by combining a thin, ultralow modulus silicone elastomer with a stretchable, strain-limiting fabric to yield a thin, breathable composite substrate. When implemented as a platform for electronics/sensors in open mesh architectures, the result is a class of device that can be strongly, but reversibly, adhered to the skin, even in locations with hair, while simultaneously offering levels of mechanical robustness that approach those of commercial athletic apparel. An appealing aspect of the ideas is that they are compatible with a wide range of previously reported stretchable active materials and devices [3] , [9] . Experimental demonstrations in various modes of physiological status monitoring and cerebral oximetry indicate an ability to form robust measurement interfaces to the body, relevant for healthcare and non-healthcare applications alike. In this paper, we present strategies for stretchable and robust integration of soft materials, thin electronic modules and elastic fabrics into systems for physiological monitoring. Experimental and theoretical studies indicate that this type of device has excellent breathability, reusability, washability, long-term usability and high adhesion. These features are not only attractive for skin-mounted devices, but also for textile-integrated electronics. 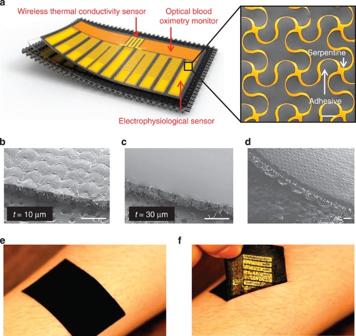Figure 1: Schematic illustration and images of rugged and stretchable electronic systems. (a) Illustrations of the various layers in a representative system, including the active electronics (~5 μm thick), an ultralow modulus elastomer coating (~100 μm thick) and a stretchable fabric (~1 mm thick; 90% nylon, 10% spandex). The active electronics layer includes a wireless thermal conductivity sensor, a blood flow monitor and an EP sensor. The magnified view shows the FS structure of part of an EP sensor, as a coloured scanning electron micrograph (SEM; gold corresponds to the conducting traces, scale bar, 100 μm). SEM images (scale bar, 1 mm) of the surface of a stretchable fabric after coating with an UL-Sil at two different thicknesses: (b) 10 μm thickness and ~200 nm roughness; (c) 30 μm thickness, ~3 nm roughness; and (d) a device transfer printed onto a substrate like the one shown inb. (e) Application and (f) detachment of the device from the skin. Rugged and breathable forms of stretchable electronics Figure 1a presents a schematic illustration of a device with a peel-away view at one of the corners to illustrate the multilayered construction. The top layer is a thin (~5 μm) electronic system consisting of metal, polymer and semiconductor materials in an open mesh architecture composed of narrow filamentary serpentine (FS) traces (widths ~60 μm) [9] , [10] . The system shown here consists of three independent functional components; a wireless thermal conductivity sensor that uses a stretchable radio frequency (RF) antenna (Cu, 3 μm thickness) coupled to an element for Joule heating (Au/Cr, 100/10 nm thickness); an optical blood oximetry monitor that uses a microscale inorganic red light emitting diode (μ-ILED; 150 × 150 μm 2 , ~2.5 μm thick; AlInGaP, with emission wavelength of 650 nm) [11] , [12] ; and an electrophysiological (EP) sensor based on three separate electrodes, each in an FS mesh geometry ( Supplementary Figs 1 and 2 ) [13] . These components, in some cases with separate additional external hardware, can be used to measure skin hydration (through thermal conductivity), blood oxygenation/perfusion (through optical scattering/absorption) and activity of the heart (electrocardiogram, ECG), muscle tissue (electromyogram, EMG), eyes (electrooculogram, EOG) or brain (electroencephalography), all via a skin interface that does not require conductive gels, penetrating micro needles, tape or straps. Figure 1: Schematic illustration and images of rugged and stretchable electronic systems. ( a ) Illustrations of the various layers in a representative system, including the active electronics (~5 μm thick), an ultralow modulus elastomer coating (~100 μm thick) and a stretchable fabric (~1 mm thick; 90% nylon, 10% spandex). The active electronics layer includes a wireless thermal conductivity sensor, a blood flow monitor and an EP sensor. The magnified view shows the FS structure of part of an EP sensor, as a coloured scanning electron micrograph (SEM; gold corresponds to the conducting traces, scale bar, 100 μm). SEM images (scale bar, 1 mm) of the surface of a stretchable fabric after coating with an UL-Sil at two different thicknesses: ( b ) 10 μm thickness and ~200 nm roughness; ( c ) 30 μm thickness, ~3 nm roughness; and ( d ) a device transfer printed onto a substrate like the one shown in b . ( e ) Application and ( f ) detachment of the device from the skin. Full size image These devices bond to an ultralow modulus silicone, (which we will refer to as UL-Sil) elastomer (Silbione RT Gel 4717 A/B, Bluestar Silicones, USA). The UL-Sil is an enabling material in this context due to its low modulus (~3.0 kPa), excellent adhesion to the skin (~1.5 kPa, measured in a peeling mode as in Supplementary Fig. 3 ), and high permeability for transepidermal water loss (~10 gh −1 m −2 at a thickness of 100 μm, measured according to ASTM E96-95, as in Supplementary Fig. 4 ). The UL-Sil exists as a thin film coating on a stretchable fabric substrate, applied by mixing a base with a curing agent, spin casting and then curing at ambient temperature. Crosslinking by polyaddition promotes the formation of an open cellular architecture by release of hydrogen gas during the reaction (penetration: 170 mm/10, DIN ISO 2137). The porosity of UL-Sil is defined by the constituent chemistry, which can include H-donors, OH-containing moieties and H-bonding agents [14] . This open, porous geometry leads to an exceptionally low modulus (much lower than the epidermis itself, ~100–200 kPa), a high degree of elasticity (able to accommodate ~250% tensile strain; Supplementary Fig. 5 ), excellent water and gas permeability and a soft, tacky but smooth surface. This last set of characteristics enables robust, reversible and non-irritating adhesion to the skin, without other materials or mechanical fixtures. The bonding, in fact, is sufficiently strong that the force required to peel a device away from the skin would, with standard embodiments of stretchable electronics, lead to catastrophic fracture of the active components. An elastic fabric of aliphatic polyamides (90%, nylon: condensation copolymers formed by reacting equal parts of a diamine and a dicarboxylic acid) and polyurethane-polyurea copolymer (10%, spandex: a long-chain synthetic polymeric fibre) addresses these and other practical challenges in ultralow modulus, skin-mounted electronics. The fabric serves as a thin (~1 mm), breathable and physically tough support that also provides a stress/strain response with strong upward curvature. In other words, the modulus increases sharply with strain above a certain threshold. Under low tensile strain, zig-zag configurations of the fibres of the fabric provide a low effective modulus. Stretching beyond a level at which the fibres are deformed into straight geometries requires significant force. These behaviours combine soft mechanics at low strains, to enable non-constraining integration with the skin, and limiting, high-modulus behaviour at high strain, to prevent fracture of the electronics. The assembly of these three mechanically and chemically distinct layers involves transfer of the electronics, fabricated in a releasable geometry on a temporary substrate, onto a piece of fabric coated with UL-Sil. High yields in transfer are possible by planarization of the fabric surface by the UL-Sil coating (for thicknesses larger than ~30 μm), as shown in Fig. 1b,c , and by its strongly adherent, tacky surface. Devices described in the following incorporate a ~100 μm thick layer of UL-Sil, as shown in Fig. 1d . 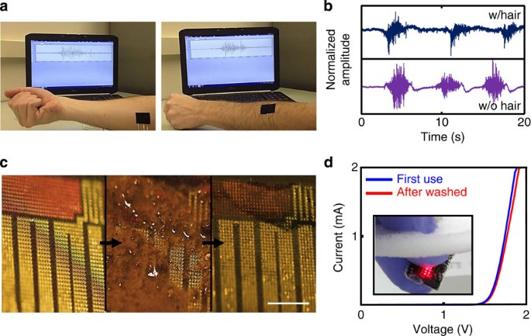Figure 2: Capabilities for applying device to the skin with hairs and washing. EMG measurement setup (a) and data (b) from inside (w/o hair) and outside of the forearm (w/hair). (c) Optical images (scale bar, 1 mm) of cleaning with soap and water: as-fabricated device (left), after contamination with dirt (center) and after washing with soap and water (right). (d) Current–voltage characteristics of an AlInGaP microscale inorganic LED module associated with the blood flow monitoring after first use and after washing. The image in the inset shows the device immersed in soapy water. Supplementary Figure 2 summarizes the fabrication steps (details in the Methods section) and the stretchable, robust mechanics of a typical device. These systems can be applied to and removed from the skin, where they adhere strongly via the soft surface of the UL-Sil, without degradation even on regions that present substantial coverage of hair ( Fig. 1e,f ). Repetitive testing indicates an ability to apply and remove a single device to and from the forearm more than ~100 times without adverse effect, either on the skin or the device ( Supplementary Fig. 6 ). Similar manipulations without the fabric substrate lead to immediate mechanical failure in the electronics, consistent with previous observations [15] . In addition to strong, reversible adhesion, this interface enables high quality recording of EP signals, as shown for the cases of EMG collected from the medial or lateral side of the right proximal forearm in Fig. 2a ; left/right frames correspond to the flexor carpi radialis/extensor carpi radialis on the inside/outside of the forearm. Notably, the signals collected in regions with hair (~20 mm long, with follicular density of around 60 per cm 2 , with about 2 mm spacing between adjacent follicular units) of Fig. 2b are comparable to those without. Also, as shown on Supplementary Fig. 7a , the adhesion to the skin decreases by only a modest amount during the course of a day. Such capabilities follow directly from the extreme conformality of the UL-Sil surface, and have significant consequences for practical use. Figure 2c demonstrates another feature that is important in this context: durability under vigorous washing with soap and water. As shown in Supplementary Fig. 7b , even after 20 washing cycles, the device retains its original shape. The results on the right in Fig. 2d illustrate that the operating characteristics of a small array of μ-ILEDs remain unchanged through a sequence of washing and drying steps. Figure 2: Capabilities for applying device to the skin with hairs and washing. EMG measurement setup ( a ) and data ( b ) from inside (w/o hair) and outside of the forearm (w/hair). ( c ) Optical images (scale bar, 1 mm) of cleaning with soap and water: as-fabricated device (left), after contamination with dirt (center) and after washing with soap and water (right). ( d ) Current–voltage characteristics of an AlInGaP microscale inorganic LED module associated with the blood flow monitoring after first use and after washing. The image in the inset shows the device immersed in soapy water. Full size image The experimental and simulation results of Fig. 3 summarize key characteristics of the materials and the composite construction that lead to these favourable device properties. As shown in Fig. 3 and Supplementary Figs 3–5 , the UL-Sil provides strong, yet non-invasive and reversible, adhesion to human skin, in a way that naturally accommodates motions of the skin as well as transepidermal water loss. In fact, the degree of adhesion to the skin, the permeability and the modulus are stronger (by ~8, shown in Fig. 3a ), higher (by ~60, shown in Fig. 3b ) and lower (by ~1,000, shown in Fig. 3c ), respectively, than those of silicones (Ecoflex, polydimethylsiloxane (PDMS) and Solaris) previously used in stretchable electronics [6] . Without the strain-limiting, stretchable fabric, however, these same favorable properties in the UL-Sil would render it impractical as a platform for the electronics. 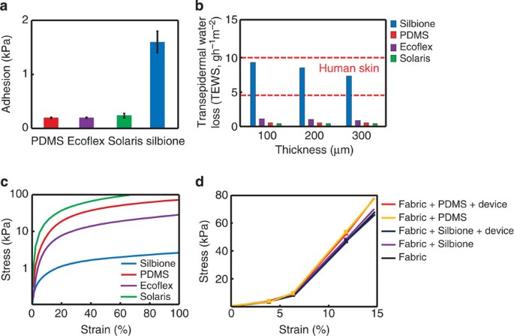Figure 3: Physical properties of composite substrate materials. (a) Comparison of adhesion strength of four common silicone elastomers to the skin. (b) Transepidermal water loss as a function of the thickness of four common silicone elastomers. (c) Stress–strain curves plotted in a semi-logarithmic scale, for four common elastomers. Although each material exhibits linear elastic response up to strains of 100%, the UL-Sil has a modulus (~3 kPa) that is nearly 1,000 times smaller than the most widely used elastomer for stretchable electronics (PDMS; ~2 MPa). (d) Stress–strain curves for stretchable fabrics with and without elastomer coatings and active electronics. The results indicate strain-limiting behaviour associated with the increasing effective modulus of the fabric with increasing strain. Also, the mechanics of the fabric dominates the mechanics of the system, for all cases. Figure 3d shows the stress/strain behaviours of the fabric, with and without elastomer coatings and mounted electronics. The findings confirm the desired behaviours. In particular, the fabric has a modulus that increases with strain, its behaviour is elastic (at the low frequencies examined here; Supplementary Fig. 5b ), and its mechanics dominate the response of the integrated system. Due to its low modulus, the UL-Sil material provides another important role in the system—it imposes only minimal constraint on motions of the FS structures in the electronic layer that occur during deformation of the entire system. 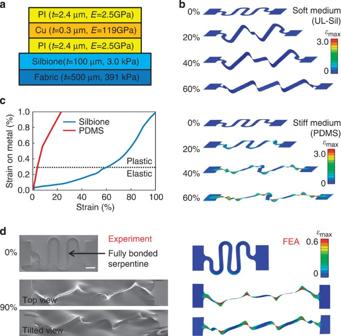Figure 4: Mechanics of materials and structures for stretchable electronics. (a) Cross-sectional illustration of representative layers in a stretchable electronic system. (b) Deformations of a FS trace and distributions of maximum principal strains in the metal computed by FEA for a system consisting of electronics/UL-Sil(3.0 kPa)/fabric and electronics/PDMS (~1–2 MPa)/fabric. (c) The computed maximum principal strains in the metal as a function of the strain applied to the entire system show enhanced stretchability with the UL-Sil material compared with PDMS. (d) Scanning electron micrographs (scale bar, 200 μm) and corresponding FEA results of undeformed and uniaxially stretched (90%) configurations of a FS trace bonded to a UL-Sil/fabric substrate. Figure 4 summarizes this unique feature and the underlying mechanics through a series of three-dimensional finite element analysis (FEA) results and experimental measurements. Figure 4 and Supplementary Figs 8 and 9 show that upon uniaxial stretching, the FS interconnects in the electronics/UL-Sil/fabric system (in Fig. 4a ) deform via twisting and in- and out-of-plane bending with little constraint imposed by the UL-Sil. By comparison, replacing the UL-Sil with PDMS significantly alters the nature of the FS deformations, as manifested by the resulting dominance of in-plane bending and wrinkling at the regions of the arcs. As a result, the maximum principal strains in the metal layers ( Fig. 4b ) are much smaller with UL-Sil than with PDMS. Quantitative accumulation of the metal strain is illustrated in Fig. 4c for both systems. For a representative yield strain of 0.3% for the copper [16] , [17] , FEA predicts an elastic-stretchability of ~60% for the electronics/UL-Sil/fabric system, which is ~15 times larger than that (~4%) of an otherwise equivalent electronics/PDMS/fabric system. Techniques based on prestrain, previously demonstrated on conventional PDMS substrates [18] , can further enhance the stretchability. Figure 4d shows an example of ~10% prestrain, in which the scanning electron micrograph images and FEA results show remarkable agreement for uniaxial strains up to 90% stretching. Here, the elastic limit increases from ~61 to ~76%. FEA indicates, in fact, that the strain in the Cu remains <0.7%, much lower than the fracture strain [19] , even under 100% stretching. Figure 3: Physical properties of composite substrate materials. ( a ) Comparison of adhesion strength of four common silicone elastomers to the skin. ( b ) Transepidermal water loss as a function of the thickness of four common silicone elastomers. ( c ) Stress–strain curves plotted in a semi-logarithmic scale, for four common elastomers. Although each material exhibits linear elastic response up to strains of 100%, the UL-Sil has a modulus (~3 kPa) that is nearly 1,000 times smaller than the most widely used elastomer for stretchable electronics (PDMS; ~2 MPa). ( d ) Stress–strain curves for stretchable fabrics with and without elastomer coatings and active electronics. The results indicate strain-limiting behaviour associated with the increasing effective modulus of the fabric with increasing strain. Also, the mechanics of the fabric dominates the mechanics of the system, for all cases. Full size image Figure 4: Mechanics of materials and structures for stretchable electronics. ( a ) Cross-sectional illustration of representative layers in a stretchable electronic system. ( b ) Deformations of a FS trace and distributions of maximum principal strains in the metal computed by FEA for a system consisting of electronics/UL-Sil(3.0 kPa)/fabric and electronics/PDMS (~1–2 MPa)/fabric. ( c ) The computed maximum principal strains in the metal as a function of the strain applied to the entire system show enhanced stretchability with the UL-Sil material compared with PDMS. ( d ) Scanning electron micrographs (scale bar, 200 μm) and corresponding FEA results of undeformed and uniaxially stretched (90%) configurations of a FS trace bonded to a UL-Sil/fabric substrate. Full size image Stretchable electronics with ultra-soft elastomer coating Experiments demonstrate that with appropriate designs, the stretchability is limited not by the electronics but by the fabric itself. 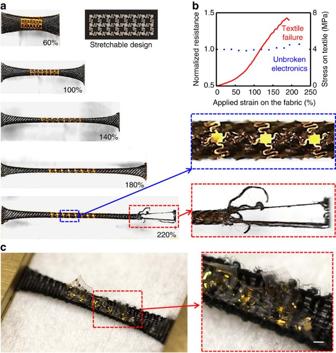Figure 5: Extreme stretchability and mechanically rugged behaviour. (a) Device integration with UL-Sil coating (E=3 kPa), Optical images of a stretchable electronic test structure (thickness ~2 μm) at increasing levels of uniaxial stretching. Magnified views of unbroken electronics (blue dotted box) and torn fabric (red dotted box) observed at an applied strain of 220%. (b) Normalized electrical resistance (leftyaxis) and applied stress (rightyaxis) as a function of tensile strain applied to the ends of the fabric substrate. (c) An optical image of the device that uses a standard formulation of silicone (PDMS, E=1 MPa), in place of the UL-Sil. The silicone tears at multiple sites and the test structures fracture at 100%. Figure 5a shows optical images of a test structure of electronics/UL-Sil/fabric (identical to that of Fig. 4a ) under various states of uniaxial deformation ( Supplementary Figs 8 and 9 ), along with data on its stress/strain and electrical/strain responses. At ~220% strain, the system begins to fail, starting with tears at the edge of the fabric near the location of clamping to the stretching fixture. The magnified images on the right highlight the location of this tearing, as well as the elastically deformed structures in the center of the device. This robust mechanics is consistent with separate measurements of electrical resistance as a function of strain, summarized in Fig. 5b . Comparative results in a system that replaces UL-Sil with PDMS appear in Fig. 5c ; here the electronics and even the underlying PDMS exhibit multiple, severe fractures and regions of delamination and plastic deformation at strains of 100%. Figure 5: Extreme stretchability and mechanically rugged behaviour. ( a ) Device integration with UL-Sil coating ( E =3 kPa), Optical images of a stretchable electronic test structure (thickness ~2 μm) at increasing levels of uniaxial stretching. Magnified views of unbroken electronics (blue dotted box) and torn fabric (red dotted box) observed at an applied strain of 220%. ( b ) Normalized electrical resistance (left y axis) and applied stress (right y axis) as a function of tensile strain applied to the ends of the fabric substrate. ( c ) An optical image of the device that uses a standard formulation of silicone (PDMS, E=1 MPa), in place of the UL-Sil. The silicone tears at multiple sites and the test structures fracture at 100%. Full size image Cerebral oximetery and wireless skin hydration monitoring The UL-Sil coating and stretchable fabric allow facile, reversible mounting of active electronics on the skin, in a way that establishes intimate interfaces for high quality measurement. Examples using the three integrated sensor modules of the Fig. 1a device, for optical blood oximetry, wireless thermal conductivity and electrophysiology, demonstrate some capabilities. Optical pulse metrology is possible with a μ-ILED that serves as a source of light and a digital camera that enables measurements of the distribution and temporal behaviour of interaction of this light with the skin. The system and demonstration results appear in Supplementary Fig. 10 . A more sophisticated application of this type of capability involves cerebral oximetry, as shown in Fig. 6 . Here, light from a μ-ILED (650 nm) diffuses into the depth of the tissue over the right prefrontal cortex; photodetection at a neighbouring region (dashed yellow box) captures scattered light, the majority of which passes unabsorbed through the scalp, the skull and the brain. Due to the optical absorption characteristics of human tissue, blood is the primary absorber of light in the red-infrared (IR) range. 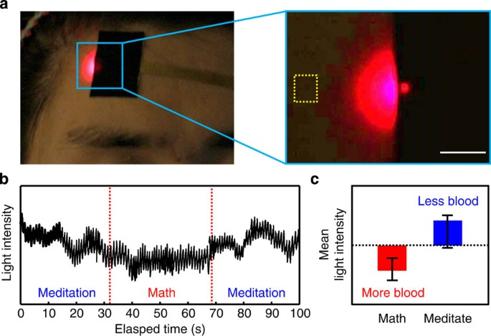Figure 6: Functional demonstration of cerebral oximetry. (a) Image of a device laminated on the skin of the forehead, with an operating μ-ILED (wavelength 650 nm) under room light illumination and in the dark. Scale bar, 1 cm. Light intensity integrated over the region indicated by the yellow dotted box of the right frame of (a), plotted as a function of time (b). (c) Scattered light intensity during mental math and rest, mean centred, smoothed with a moving window and averaged over time for each condition. Error bars denote +/−1 s.d. of the signal over time in each condition. Reduced intensity during mental activity is consistent with increased light absorption induced by additional blood flow in the cerebral cortex. Figure 6b shows results recorded while the participant alternates between resting and performing mental math exercises with their eyes closed (counting backwards by 7 from 200). The data are mean centred for each condition, and then smoothed by applying a 650 ms moving window average to eliminate the influence of the heart beat. The estimated cerebral blood flow is then averaged over time to yield the estimated average blood flow in each condition shown in Fig. 6c . As expected [20] , [21] , the measurements indicate increased blood flow during mental math compared with meditation. Figure 6: Functional demonstration of cerebral oximetry. ( a ) Image of a device laminated on the skin of the forehead, with an operating μ-ILED (wavelength 650 nm) under room light illumination and in the dark. Scale bar, 1 cm. Light intensity integrated over the region indicated by the yellow dotted box of the right frame of ( a ), plotted as a function of time ( b ). ( c ) Scattered light intensity during mental math and rest, mean centred, smoothed with a moving window and averaged over time for each condition. Error bars denote +/−1 s.d. of the signal over time in each condition. Reduced intensity during mental activity is consistent with increased light absorption induced by additional blood flow in the cerebral cortex. Full size image Capabilities in wireless operation are important for many envisioned applications. A simple example of controlled, wireless heating via far field exposure to RF radiation appears in IR images in Fig. 7a,b ; Supplementary Fig. 11 . Here, a stretchable RF antenna in a dipole geometry (30 mm for each branch, for operation at ~2.4 GHz in air, and at ~0.9 GHz on skin, as in Fig. 7c ) with a FS mesh layout (Cu traces, 3 μm thick and 10 mm wide, encapsulated above and below with PI) absorbs incident RF energy. The resulting induced current oscillates at the operating frequency, to create Joule heating in a resistive element (Au/Cr, 100/15 nm thick) that has a much higher resistance (~500 Ω) than the antenna (~5 Ω). This element appears as bright spots in the centres of the dashed yellow boxes in Fig. 7a,b . Time-dependent measurements of the temperature, recorded electrically or through analysis of the IR images, capture dynamics of heating and cooling that can yield quantitative values for the thermal conductivity of the skin. The analysis involves characterizing the rise (and/or fall) times from data like those in Fig. 7d and applying transient plane source analysis [22] . 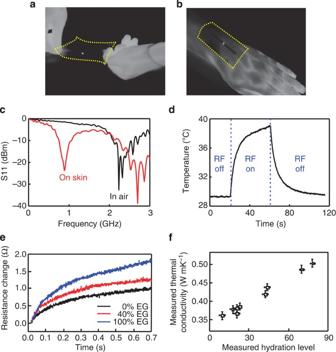Figure 7: Wireless evaluation of skin thermal properties. IR images of a wireless heating device, collected during exposure to RF energy, in a free-standing state (a) and mounted on the wrist area (b). (c)S11coefficient measured from the wireless heating element, evaluated in air and on human skin. (d) Transient control of temperature on the skin using the wireless heating element, and measured using an IR camera. The temporal behaviour during heating and during cooling define the thermal conductivity of the skin and, therefore, its hydration state. (e) Representative resistance changes during transient heat pulse measurements on three different calibration solutions. (f) Transient heat source measurements, converted to thermal conductivity, on skin. The hydration level corresponds to results of measurement with a commercially available skin moisture meter (Delfin, Finland), based on skin impedance. Error bars correspond to average s.d. values during repeated calibration measurements. Figure 7e and Supplementary Fig. 12 show results of measurements of calibration standards, to verify the approach. The conductivity correlates well to skin hydration, a physiological parameter of general interest, as illustrated in Fig. 7f through comparison with measurements using a commercial impedance-based meter (Delfin, Finland). Figure 7: Wireless evaluation of skin thermal properties. IR images of a wireless heating device, collected during exposure to RF energy, in a free-standing state ( a ) and mounted on the wrist area ( b ). ( c ) S 11 coefficient measured from the wireless heating element, evaluated in air and on human skin. ( d ) Transient control of temperature on the skin using the wireless heating element, and measured using an IR camera. The temporal behaviour during heating and during cooling define the thermal conductivity of the skin and, therefore, its hydration state. ( e ) Representative resistance changes during transient heat pulse measurements on three different calibration solutions. ( f ) Transient heat source measurements, converted to thermal conductivity, on skin. The hydration level corresponds to results of measurement with a commercially available skin moisture meter (Delfin, Finland), based on skin impedance. Error bars correspond to average s.d. values during repeated calibration measurements. Full size image Multiple site EP sensing The materials and device construction allow continuous use in realistic scenarios. 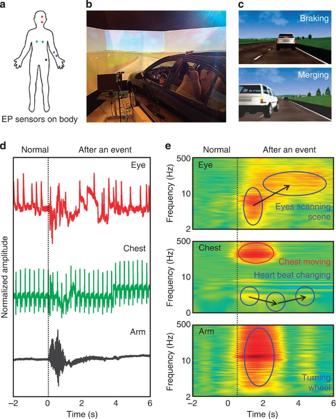Figure 8: EP monitoring of a human subject in a driving simulator. (a) Schematic illustration of the locations of the EP sensors on the body. (b) Configuration of a driving simulator that uses eight large screens surrounding a full-scale test vehicle to provide a realistic, but virtual, driving experience. A driver wearing EP sensors is in the simulator car. (c) Representative driving scenarios for EP monitoring. (d) Typical EP signals recorded during unexpected braking and merging events. (e) Spectrographs of the EP signals. A total 11 braking and 12 merging events occurred during 40 min, while the multiple sensors continuously collected EP data. Figure 8 ; Supplementary Fig. 13 present examples of EP measurements on a human subject engaged in an immersive, full-scale driving simulator. Here, as shown in Fig. 8a,b , several sensors placed on multiple sites of the body simultaneously record EOG, for eye movements, EMG, for movements of the chest/arms and ECG, with a ground electrode placed on the left hip. The signal analysis procedures appear in the Methods section. As the participant drives for 45 min under busy highway conditions with 100 other cars, some of which intermittently merge into or brake in front of the driver’s path, the EP information reveals various responses, as shown in Fig. 8c . Figure 8d shows normalized EOG (red), ECG/EMG (green) and EMG (blue) time-locked to a representative braking event at t =0. The data show that the driver reacts with quick eye movements to the car, muscle movements to move the steering wheel and a decelerated heart rate in response to this challenging driving event. Figure 8e shows the average event-related spectrogram for EOG, ECG and EMG for all 21 braking and merging events, computed with a 4,096-point moving window discrete Fourier transform of the 20 s before and after the braking events. For each trial, subtraction of the average spectra from 2–5 s before the braking event isolates evoked changes in physiology. The EOG activity indicates a sharp increase in eye movements after the event, followed by a sustained high frequency set of movements. A device on the chest measures both an increase in EMG activity of the chest muscles in response to the braking event, as well as a peak at the frequency of the heart rate that decreases in the period following a braking event. The EMG activity indicates a sustained increase in high frequency muscle activity as the participant moves their arms and the steering wheel in response to the braking car. Due to the thin, elastic construction of the devices, and their soft, reversible adhesion onto the skin, all of these measurements occur without measurable effect on natural response. Figure 8: EP monitoring of a human subject in a driving simulator. ( a ) Schematic illustration of the locations of the EP sensors on the body. ( b ) Configuration of a driving simulator that uses eight large screens surrounding a full-scale test vehicle to provide a realistic, but virtual, driving experience. A driver wearing EP sensors is in the simulator car. ( c ) Representative driving scenarios for EP monitoring. ( d ) Typical EP signals recorded during unexpected braking and merging events. ( e ) Spectrographs of the EP signals. A total 11 braking and 12 merging events occurred during 40 min, while the multiple sensors continuously collected EP data. Full size image The results presented here indicate that heterogeneous integration of semiconductors, metals and polymer dielectrics in filamentary, open mesh designs for active electronics and sensors, with ultralow modulus, permeable elastomer coatings for conformal skin adhesion, on breathable, stretchable fabrics as rugged substrates yields an attractive architecture for skin-mounted devices. The UL-Sil and the fabric are the critical materials components in these systems. The former provides a smooth, conformable surface for strong adhesion and reversible bonding to the skin, even in regions with substantial hair, and the electronics, in a manner that imposes minimal mechanical constraints on their motion. The latter provides a robust, strain limiting support for the UL-Sil, whose ultralow modulus and strong adhesion would otherwise prevent its use in practical applications. These two materials form a composite substrate that is compatible with natural processes of transepidermal water loss, and offers capability for use not only with the types of active components described here, but also with stretchable conductors, organic semiconductors and low-dimensional materials such as carbon nanotubes, silver nanowires and graphene, reported elsewhere [23] , [24] , [25] , [26] . Although experiments, modelling results and demonstration experiments indicate many appealing characteristics, there are additional opportunities for optimizing of properties of this substrate, through development of engineered fabrics and tailored elastomer coatings. Device fabrication Spin casting formed thin layers of polydimethylsiloxane (PDMS; 10 μm in thickness, Dow Corning, USA) and polyimide (PI; 1.2 μm in thickness, Sigma-Aldrich, USA) on a temporary glass substrate. Two μ-ILEDs prepared according to previously described procedures [11] were transfer printed onto the PI. Thermally curing the PI (2 h at 210 °C) yielded strong bonds to μ-ILEDs. The wireless heater and EP sensors used photolithographically patterned bi-layers of Cr (15 nm)/Au (100 nm) formed by sputter deposition (AJA sputter, 150 W/50 W). The RF antenna used Cu (3 μm) by electron beam evaporation. Spin casting a layer of PI (2,000 r.p.m.) passivated and isolated the devices. Reactive ion etching (20 sccm O 2 , 200 W, 200 mTorr) through a photolithographically patterned hard mask (Cu, 100 nm thick) removed the PI in the regions between the devices. A water soluble tape (3 M, USA) allowed retrieval of the completed patterns from the glass substrate and delivery to an adhesive (UL-Sil or PDMS)-coated stretchable textile substrate. Finite element analysis Three-dimensional FEA techniques allowed investigation of the mechanics of devices on UL-Sil/textile or PDMS/textile substrates. Eight-node three-dimensional solid elements and four-node shell elements were used for the bi-layer substrate and serpentine interconnect, respectively, with refined meshes to ensure the accuracy. Displacement-type boundary conditions were assigned to the side surfaces of substrate to apply to different levels of stretching. The Young’s modulus ( E ) and Poisson ratio ( ν ) of the materials used in the simulations include E Cu =119 GPa and ν Cu =0.34 for copper; E PI =2.5 GPa and ν PI =0.34 for PI; E Textile =391 kPa and ν Textile =0.40 for textile (approximated, for purposes of simulation, to have linear elastic properties); E UL-Sil =3.0 kPa and ν Silbione =0.49 for UL-SIl; and E PDMS =1 MPa and ν PDMS =0.49 for PDMS. Wireless heater system A network analyser (E5602, Agilent Technologies, USA) with calibration kit (85033E, Agilent Technologies, USA) enabled measurement of the return loss ( S 11 ) and the resonance frequency of the RF antennas. RF signals precisely controlled with an analogue signal generator (N5181A, Agilent Technologies, USA), an amplifier (1119, EMPOWER RF System, USA), a DC power supply (U8031A, Agilent Technologies, USA). Directional antenna with 10.5 dBi gain (204411, Wilson Electronics, USA) and an RF power meter (43, Bird Technologies, USA) were used to expose a wireless heater laminated on the arm (~2 kg) of an adult human subject. The power levels (<10 W) were maintained below FCC guidelines (8 W kg −1 for partial body irradiation). The temperature distributions were measured using an IR camera (A655SC, FLIR). Measurements of skin hydration Thermal conductivity was determined by analysing the time constant for the rise in temperature determined using a resistive detector after ~0.7 s of Joule heating. Conversion to thermal conductivity relied on calibration data collected from aqueous ethylene glycol solutions with known thermal conductivities, as shown in Supplementary Fig. 12 . Measurements of EP signals All experiments involving human subjects were conducted under approval from Institutional Review Board at the University of Illinois at Urbana-Champaign (protocol number: 13,229). There were six subjects (age: 21–32, all males). Research was carried out with informed consent. For the data of Fig. 2b , the right wrist was extended every 5 s. Data were digitized at 256 Hz, with a 60 Hz notch filter to eliminate electrical noise. Data were amplified and transmitted wirelessly to a recording PC using an amplifier (CleveMed, USA) as the difference in voltage between two EP sensors on the device, spaced 40 mm apart. A ground electrode was placed over a bony protrusion of the right lateral ankle. The mean value was subtracted from original signal, and the data were divided by their maximum value to compute normalized EMG amplitude. Supplementary Movie 1 demonstrates stretchability, reusability, washability of fabric-based stretchable electronic devices. EMG measurements show capabilities for mounting on regions of the skin with hair. Optical measurements of oximetry An analysis programme stabilized all frames of video collected with a digital camera by template correlation with the first frame, and then determined the time variation of the average light intensity evaluated inside a region of interest (dotted yellow box) for only the red RGB channel. A band-pass filter between 0.5 and 3 Hz removed high frequency noise and low frequency drifts in the data. A discrete Fourier transform of the filtered signal revealed the beat rate. For cerebral oximetry, a 3-mm diameter fibre-optic bundle was held flush against the head to collect light and transmit it to a photomultiplier tube detector (Imagent, USA). Evaluations in the driving simulator The experiments were conducted in the Beckman Institute Illinois Simulator Laboratory. A total of eight textile EP sensors were placed on the skin at various locations across the body. EOG data were recorded from bipolar electrodes placed superior (and slightly medial) and inferior (and slightly lateral) to the participant’s left eye, in a position sensitive to both horizontal and vertical eye movements. ECG data were recorded from bipolar electrodes placed over the most medial areas of the left and right fourth intercostal spaces. EMG data were recorded from bipolar electrodes over the proximal left forearm over the flexor carpi radialis muscle. All three pairs of bipolar textile electrodes were used simultaneously with a common ground electrode placed on the human subject’s left hip. Voltage differences between bipolar pairs of textile electrodes were amplified and digitized with a Neuroscan SynAmps 32-Channel amplifier at 2,000-Hz with a 0.1–1,000 Hz online band-pass filter to remove slow drifts and high frequency non-physiological noise, and a 60-Hz notch filter to attenuate electrical line noise from the simulator. The participant drove in a Hyperdrive driving simulator for 45 min in a busy highway driving scenario with 100 other cars. Cars intermittently merged into the driver’s path, or braked in front of the driver, to simulate challenging driving scenarios. The normalized EOG (red), ECG (green) and EMG (blue) activity time-locked to the onset of a single braking event at time (0). In response to this challenging driving event, the driver reacted with quick eye motions to the car, muscle activity to move the steering wheel and a decelerated heart rate. The average event-related spectrograms for EOG, ECG and EMG corresponds to responses for all 21 braking and merging events, computed with a 4,096-point moving window DFT of the 20 s before and after the braking events. For each trial, the average spectra from 5–2 s before the braking event were subtracted from each time point to isolate the evoked changes in physiology from the event. How to cite this article : Jang, K.-I. et al. Rugged and breathable forms of stretchable electronics with adherent composite substrates for transcutaneous monitoring. Nat. Commun. 5:4779 doi: 10.1038/ncomms5779 (2014).